Heat shock factor-1 influences pathological lesion distribution of polyglutamine-induced neurodegeneration A crucial feature of adult-onset neurodegenerative diseases is accumulation of abnormal protein in specific brain regions, although the mechanism underlying this pathological selectivity remains unclear. Heat shock factor-1 is a transcriptional regulator of heat shock proteins, molecular chaperones that abrogate neurodegeneration by refolding and solubilizing pathogenic proteins. Here we show that heat shock factor-1 expression levels are associated with the accumulation of pathogenic androgen receptor in spinal and bulbar muscular atrophy, a polyglutamine-induced neurodegenerative disease. In heterozygous heat shock factor-1 -knockout spinal and bulbar muscular atrophy mice, abnormal androgen receptor accumulates in the cerebral visual cortex, liver and pituitary, which are not affected in their genetically unmodified counterparts. The depletion of heat shock factor-1 also expands the distribution of pathogenic androgen receptor accumulation in other neuronal regions. Furthermore, lentiviral-mediated delivery of heat shock factor-1 into the brain of spinal and bulbar muscular atrophy mice topically suppresses the pathogenic androgen receptor accumulation and neuronal atrophy. These results suggest that heat shock factor-1 influences the pathological lesion selectivity in spinal and bulbar muscular atrophy. Heat shock proteins (Hsps), including Hsp70 and Hsp40, are stress-induced molecular chaperones that have important roles in maintaining correct folding, the assembly of newly synthesized proteins and the intracellular transport of proteins [1] , [2] . There are various lines of evidence indicating that Hsps abrogate neurodegeneration by refolding and solubilizing pathogenic proteins [3] , [4] . Particularly, Hsp70 facilitates the proteasomal degradation of abnormal proteins and thereby ameliorates neuronal damage in cellular and animal models of adult-onset neurodegenerative disorders, including Alzheimer’s disease, amyotrophic lateral sclerosis and Huntington’ disease (HD) [5] , [6] , [7] and other polyglutamine diseases caused by the expansion of a genomic CAG repeat [8] , [9] , [10] . Among several molecules that control the expression of Hsps, heat shock factor-1 (Hsf-1) is shown to strongly regulate the expression of Hsp70 by activating its promoter [11] , [12] . To develop effective treatments for neurodegenerative disorders, it is important to elucidate the molecular mechanism by which only specific cells are affected, despite the broad expression of the disease-causing mutant genes. The selectivity of the pathogenic lesions in neurodegenerative diseases may be influenced by several factors. For example, the length of the CAG triplet repeat in the causative gene influences the distribution of pathological lesions of spinocerebellar ataxia type 7 and dentatorubral pallidoluysian atrophy [13] , [14] . Given that the length of the polyglutamine tract increases the propensity of the protein to aggregate, the pathological lesion selectivity of spinocerebellar ataxia type 7 appears to be influenced by the biological properties of the causative protein [15] . Alternatively, the expression of molecules that interact with the disease-causing proteins, such as PQBP-1 and Rhes, is also associated with the distribution of selective neuronal cell loss in polyglutamine diseases [16] , [17] . Furthermore, transcriptional factors such as nuclear transcription factor Y subunit alpha (NF-YA) and p53 were shown to, at least partially, determine the vulnerability of cells to polyglutamine-expanded proteins by regulating the expression of Hsps in cellular models of HD [18] , [19] . The accumulation of polyglutamine-expanded proteins is detected histopathologically as diffuse nuclear staining or as intraneuronal inclusion bodies, the distribution of which corresponds to that of pathological involvement and symptomatic phenotypes [20] , [21] . The intranuclear accumulation of disease-causing misfolded proteins is thought to trigger neurodegeneration by various mechanisms such as transcriptional dysregulation, impairment of axonal transport and mitochondrial dysfunction [22] , [23] , [24] . This view is supported by animal studies showing that the prevention of pathogenic protein accumulation successfully rescues the phenotype in model mice of polyglutamine diseases [25] , [26] , [27] , [28] . Here, we investigated the role of Hsf-1 in pathogenic lesion selectivity in spinal and bulbar muscular atrophy (SBMA), an adult-onset motor neuron disease caused by the expansion of a CAG repeat in the gene coding androgen receptor (AR) [29] , [30] , [31] . This disease affects susceptible regions, such as spinal anterior horn, brainstem and pancreas, despite the ubiquitous expression of the causative protein [32] . In the present study, we found that the heterozygous knockout of Hsf-1 in SBMA model mice led to the extended distribution of pathogenic AR accumulation in neuronal and non-neuronal tissues as well as exacerbated neuromuscular phenotype, whereas the lentiviral overexpression of HSF-1 locally precludes pathogenic AR accumulation and neuronal atrophy in the brain of the SBMA mice. Hsf-1 levels are associated with pathogenic AR accumulation To examine whether the expression levels of Hsf-1 are associated with the distribution of pathogenic AR accumulation in SBMA, we performed immunohistochemistry on the central nervous system (CNS) of a transgenic SBMA mouse model carrying human AR with 97 CAGs (AR-97Q). In this model animal, the full-length human AR was expressed ubiquitously ( Supplementary Fig. S1a ). The results showed that low expression levels of Hsf-1 were associated with a high frequency of pathogenic AR accumulation ( Fig. 1a ). For example, the accumulation of pathogenic AR is frequently observed in spinal motor neurons that show weak immunoreactivity for Hsf-1. In contrast, neurons in the cerebral cortex and striatum, most of which are Hsf-1-positive, were rarely stained with 1C2, a specific antibody against the expanded polyglutamine tract. In the cerebellum of AR-97Q mice, there was a scarce accumulation of pathogenic AR in Purkinje cells, where Hsf-1 was expressed at a high level. Conversely, there were abundant 1C2-positive cells in the cerebellar granular cell layer, which showed scarce immunoreactivity for Hsf-1 ( Fig. 1a ). There was little difference in the expression pattern of Hsf-1 between AR-97Q and wild-type mice, except for the spinal anterior horn, where the nuclear expression of Hsf-1 was decreased in AR-97Q mice compared with wild-type mice ( Fig. 1a ). Quantitative analysis of the relationship between the expression levels of Hsf-1 and the frequency of 1C2-positive cells in various parts of the CNS confirmed that higher expression levels of Hsf-1 are associated with the reduced accumulation of pathogenic AR ( Fig. 1b ). This relationship, however, was not clearly observed for Nfya, p53, TATA box-binding protein (Tbp) or Sp1, which are other potential inducers of Hsp70 ( Supplementary Fig. S1b,c ). These findings led us to focus on Hsf-1 as a possible regulator of the pathogenic lesion selectivity, especially in the CNS, of the SBMA model mouse. 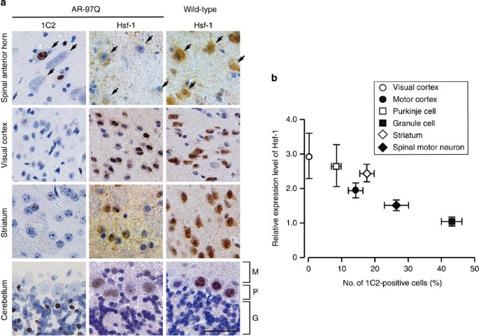Figure 1: Hsf-1 expression is associated with pathogenic AR accumulation. (a) Immunohistochemistry for Hsf-1 and expanded polyglutamine (1C2) in the spinal anterior horn, visual cortex, striatum and cerebellum from wild-type and AR-97Q mice (13 weeks old). Arrows indicate motor neurons within the spinal anterior horn. M, molecular layer; P, Purkinje cell layer; G, granular layer. (b) Quantification of the relationship between the nuclear immunoreactivity of Hsf-1 and the frequency of 1C2-positive cells in different parts of the CNS. More than 500 neurons in each part from three brains were analysed (b). Error bars indicate s.e.m. (b). Scale bars, 50 μm (a). Figure 1: Hsf-1 expression is associated with pathogenic AR accumulation. ( a ) Immunohistochemistry for Hsf-1 and expanded polyglutamine (1C2) in the spinal anterior horn, visual cortex, striatum and cerebellum from wild-type and AR-97Q mice (13 weeks old). Arrows indicate motor neurons within the spinal anterior horn. M, molecular layer; P, Purkinje cell layer; G, granular layer. ( b ) Quantification of the relationship between the nuclear immunoreactivity of Hsf-1 and the frequency of 1C2-positive cells in different parts of the CNS. More than 500 neurons in each part from three brains were analysed ( b ). Error bars indicate s.e.m. ( b ). Scale bars, 50 μm ( a ). Full size image Previous studies showed that AR-97Q mice show pathogenic AR aggregation in non-neuronal tissues, such as the heart, lung, pancreas and skeletal muscle, in addition to the CNS [25] . To examine whether the expression levels of Hsf-1 are also associated with pathogenic AR accumulation outside the CNS, we performed immunohistochemistry using anti-Hsf-1 and 1C2 antibodies on non-neuronal tissues of the AR-97Q mice. The results demonstrated that a similar relationship as seen in CNS was observed in the pancreas, liver and testis. There was unequivocal pathogenic AR accumulation in the pancreas, where Hsf-1 is expressed at a low level ( Supplementary Fig. S1d ). In contrast, no visible pathogenic AR accumulation was observed in the liver or testis, where Hsf-1 is expressed at a relatively high level ( Supplementary Fig. S1d ). We further verified this relationship in autopsied specimens from SBMA patients. 1C2-positive cells were frequently detected in spinal motor neurons and pancreatic islet cells, where HSF-1 is expressed at a low level, compared with control subjects. In contrast, there were no 1C2-stained cells in the neuronal and non-neuronal tissues in which HSF-1 was expressed at a high level ( Supplementary Fig. S2a,b ). Taken together, these results indicate that high expression levels of Hsf-1 are associated with reduced pathogenic AR accumulation in neuronal and non-neuronal tissues of the SBMA mouse model and SBMA patients. Hsf-1 depletion expands distribution of AR accumulation To clarify whether low expression levels of Hsf-1 have a causative role in the accumulation of pathogenic AR in vivo , we depleted Hsf-1 in AR-97Q mice by crossing them with heterozygous Hsf-1 -knockout mice [33] . As Hsf-1 -null AR-97Q (AR-97Q Tg/−, Hsf-1 −/−) mice were not obtained, presumably owing to their early death during embryonic development, we performed immunohistochemistry on various tissues from wild-type (AR-97Q−/−, Hsf-1 +/+), AR-97Q (AR-97Q Tg/−, Hsf-1 +/+) and heterozygous Hsf-1 -knockout AR-97Q (AR-97Q Tg/−, Hsf-1 +/−) mice, to examine whether Hsf-1 inactivation expands the distribution of pathogenic AR accumulation. The nuclear accumulation of pathogenic AR is not detected in the liver and pituitary gland of AR-97Q mice, even at an advanced stage ( Supplementary Fig. S3 ). Surprisingly, we observed the nuclear accumulation of pathogenic AR in the liver of the heterozygous Hsf-1 -knockout SBMA mice ( Fig. 2a ). Quantitative analysis showed that 1.40±0.35% (1.0–2.1) of hepatocytes were positive for 1C2 in the Hsf-1 -depleted AR-97Q mice, while no positive cells were observed in the AR-97Q mice ( n =3 per group). To confirm the effects of Hsf-1 depletion on the metabolism of pathogenic AR, we performed immunoblotting of the liver samples using an anti-AR antibody. The results revealed that the expression level of AR monomer, which appears to be one of the toxic species of polyglutamine protein [34] , was increased by the heterozygous knockout of Hsf-1 in the liver of AR-97Q mice ( Fig. 2b ). Insoluble high-molecular-weight AR complexes, which may have a protective property, were not detected in the liver of either type of mice, presumably because of the relatively low expression levels of AR in this tissue. 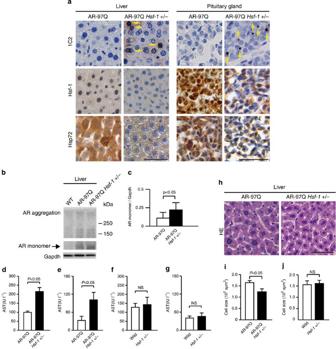Figure 2: Pathogenic AR accumulates in the liver and pituitary gland of heterozygousHsf-1-knockout AR-97Q mice. (a) Immunohistochemistry of AR-97Q andHsf-1-knockout AR-97Q mice using anti-Hsf-1, anti-Hsp72 and anti-polyglutamine (1C2) antibodies (13 weeks old). TheHsf-1-knockout AR-97Q mice showed the nuclear accumulation of pathogenic AR (yellow arrows) and decreased levels of Hsf-1 and Hsp72, an inducible form of Hsp70, in the liver and pituitary gland. (b) Immunoblotting for AR in wild-type, AR-97Q andHsf-1-knockout AR-97Q mice (13 weeks old). (c) Quantification of immunoblotting revealed that the expression levels of AR monomer were upregulated in the liver of heterozygousHsf-1-knockout AR-97Q mice. Unpairedt-test,n=3. (d–g) Blood tests revealed that the liver enzyme levels, including aspartate aminotransferase (AST) (d) and alanine aminotransferase (ALT) (e), were elevated in heterozygousHsf-1-knockout AR-97Q mice compared with AR-97Q mice (13 weeks old). There were no significant differences in the levels of AST (f) and ALT (g) between wild-type and heterozygousHsf-1-knockout mice (13 weeks old). (h) Haematoxylin–eosin staining of the liver of heterozygousHsf-1-knockout and genetically unmodified AR-97Q mice (13 weeks old). (i) Quantitative analysis showed that the size of hepatocytes was reduced in heterozygousHsf-1-knockout AR-97Q mice compared with AR-97Q mice. (j) Depletion ofHsf-1did not alter the size of hepatocytes in wild-type mice. Unpairedt-test (n=4) (d–g). More than 1,000 cells from three livers were analysed in each group, unpairedt-test. (i,j). Error bars indicate s.e.m. (c–g,i,j). Scale bars, 50 μm (a,h). NS, not significant. Figure 2: Pathogenic AR accumulates in the liver and pituitary gland of heterozygous Hsf-1 -knockout AR-97Q mice. ( a ) Immunohistochemistry of AR-97Q and Hsf-1 -knockout AR-97Q mice using anti-Hsf-1, anti-Hsp72 and anti-polyglutamine (1C2) antibodies (13 weeks old). The Hsf-1 -knockout AR-97Q mice showed the nuclear accumulation of pathogenic AR (yellow arrows) and decreased levels of Hsf-1 and Hsp72, an inducible form of Hsp70, in the liver and pituitary gland. ( b ) Immunoblotting for AR in wild-type, AR-97Q and Hsf-1 -knockout AR-97Q mice (13 weeks old). ( c ) Quantification of immunoblotting revealed that the expression levels of AR monomer were upregulated in the liver of heterozygous Hsf-1 -knockout AR-97Q mice. Unpaired t -test, n =3. ( d – g ) Blood tests revealed that the liver enzyme levels, including aspartate aminotransferase (AST) ( d ) and alanine aminotransferase (ALT) ( e ), were elevated in heterozygous Hsf-1 -knockout AR-97Q mice compared with AR-97Q mice (13 weeks old). There were no significant differences in the levels of AST ( f ) and ALT ( g ) between wild-type and heterozygous Hsf-1 -knockout mice (13 weeks old). ( h ) Haematoxylin–eosin staining of the liver of heterozygous Hsf-1 -knockout and genetically unmodified AR-97Q mice (13 weeks old). ( i ) Quantitative analysis showed that the size of hepatocytes was reduced in heterozygous Hsf-1 -knockout AR-97Q mice compared with AR-97Q mice. ( j ) Depletion of Hsf-1 did not alter the size of hepatocytes in wild-type mice. Unpaired t -test ( n =4) ( d – g ). More than 1,000 cells from three livers were analysed in each group, unpaired t -test. ( i , j ). Error bars indicate s.e.m. ( c – g , i , j ). Scale bars, 50 μm ( a , h ). NS, not significant. Full size image To assess whether the accumulation of pathogenic AR due to Hsf-1 depletion impairs liver function, we performed histology and blood tests on each mouse group. The serum levels of liver enzymes, such as aspartate aminotransferase and alanine aminotransferase, which are indicative of liver dysfunction, were significantly elevated in heterozygous Hsf-1 -knockout AR-97Q mice compared with the genetically unmodified AR-97Q mice ( Fig. 2d ), while this was not the case for wild-type mice ( Fig. 2f ). Furthermore, immunohistochemistry demonstrated that the liver became atrophied in the heterozygous Hsf-1 -knockout AR-97Q mice, but not in their wild-type counterparts ( Fig. 2h–j ). Similarly, pathogenic AR accumulation was also detected in the pituitary gland of the heterozygous Hsf-1 -knockout SBMA mice ( Fig. 2a ). A total of 0.67±0.17% (0.5–1.0) of the cells in the pituitary gland of the heterozygous Hsf-1 -knockout AR-97Q mice exhibited the nuclear accumulation of pathogenic AR, although there were no 1C2-positive cells in the pituitary gland of genetically unmodified AR-97Q mice ( n =3 per group). These findings indicate that Hsf-1 prevents the accumulation of pathogenic AR in the liver and pituitary gland of AR-97Q mice. A similar phenomenon was observed in certain parts of the CNS in AR-97Q mice. Interestingly, the accumulation of pathogenic AR was detected in the cerebral visual cortex of heterozygous Hsf-1 -knockout SBMA mice ( Fig. 3a ), where the accumulation of pathogenic AR was not observed in the AR-97Q mice, even at an advanced stage ( Supplementary Fig. S3 ). Furthermore, the heterozygous knockout of Hsf-1 also augmented the accumulation of pathogenic AR in spinal motor neurons and Purkinje cells as well as the neurons of the striatum through Hsp70 downregulation ( Fig. 3a and Supplementary Fig. S4a ). Quantitative analysis of the change in the relationship between the Hsf-1 expression levels and the frequency of 1C2-positive cells confirmed that the accumulation of pathogenic AR was significantly increased by the heterozygous depletion of Hsf-1 ( Fig. 3b–e ). Although pathogenic AR mainly accumulated in the fifth and sixth layers of the cerebral motor cortex in the AR-97Q mice, where the expression levels of Hsf-1 are relatively lower than in the other layers, the distribution of pathogenic AR accumulation was expanded to the second and third layers in the heterozygous Hsf-1 -knockout AR-97Q mice ( Fig. 3f ). The heterozygous knockout of Hsf-1 also altered the distribution and frequency of pathogenic AR accumulation in neuronal and non-neuronal tissues in the AR-97Q mice ( Supplementary Fig. S4b and Supplementary Table S1 ). To verify the impact of Hsf-1 depletion upon the pathogenic AR aggregations, we next analysed immunoblots of the spinal cord, cerebral cortex, striatum and cerebellum using an anti-AR antibody. The findings showed that the amount of smearing AR protein, which corresponds to the toxic oligomers, was increased by the heterozygous depletion of Hsf-1 in each part of the CNS of the AR-97Q mice ( Fig. 3g–i ). These findings suggest that Hsf-1 expression levels influence the degree of pathogenic AR accumulation in the SBMA mouse model. 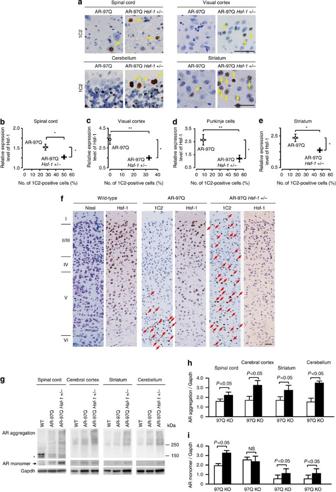Figure 3: Augmentation of pathogenic AR accumulation in the CNS ofHsf-1-knockout AR-97Q mice. (a) Immunohistochemistry for 1C2, Hsf-1 and Hsp72 in AR-97Q andHsf-1-knockout AR-97Q mice (13 weeks old). Pathogenic AR (yellow arrows) accumulated in the cerebral visual cortex of heterozygousHsf-1-knockout SBMA mice where the accumulation of pathogenic AR was not observed in the AR-97Q mice. (b–e) The change in the relationship between the expression levels of Hsf-1 and the frequency of 1C2-positive neurons in the spinal anterior horn (b), cerebral visual cortex (c), Purkinje cells of the cerebellum (d) and striatum (e). (f) Immunohistochemistry for Hsf-1 and 1C2 in the cerebral motor cortex of AR-97Q andHsf-1-knockout AR-97Q mice (13 weeks old). In AR-97Q mice, 1C2-positive cells were observed in the fifth layer of the cerebral motor cortex, where the expression levels of Hsf-1 were relatively lower than in the other layers. The distribution of pathogenic AR accumulation (red arrows) was expanded to the second and third layers of the cerebral motor cortex in heterozygousHsf-1-knockout AR-97Q mice. (g) Immunoblotting for AR in wild-type, AR-97Q andHsf-1-knockout AR-97Q mice (13 weeks old). Pathogenic AR oligomers are indicated by a smear from the top of the gel. *Nonspecific bands. (h) Quantitative analysis of immunoblots using densitometry indicated that the expression levels of abnormal AR protein complexes in the spinal cord, cerebral cortex, striatum and cerebellum were upregulated in heterozygousHsf-1-knockout AR-97Q mice compared with AR-97Q mice. (i) Quantification of immunoblotting revealed that the expression levels of AR monomer were upregulated in the spinal cord, striatum and cerebellum of heterozygousHsf-1-knockout AR-97Q mice. *P<0.05, **P<0.01 by unpairedt-test. More than 500 neurons from three brains were analysed in each group (b–e). Unpairedt-test (n=3) (h,i). Error bars indicate s.e.m. (b–e,h,i). Scale bars, 50 μm (a). NS, not significant. Figure 3: Augmentation of pathogenic AR accumulation in the CNS of Hsf-1 -knockout AR-97Q mice. ( a ) Immunohistochemistry for 1C2, Hsf-1 and Hsp72 in AR-97Q and Hsf-1 -knockout AR-97Q mice (13 weeks old). Pathogenic AR (yellow arrows) accumulated in the cerebral visual cortex of heterozygous Hsf-1 -knockout SBMA mice where the accumulation of pathogenic AR was not observed in the AR-97Q mice. ( b – e ) The change in the relationship between the expression levels of Hsf-1 and the frequency of 1C2-positive neurons in the spinal anterior horn ( b ), cerebral visual cortex ( c ), Purkinje cells of the cerebellum ( d ) and striatum ( e ). ( f ) Immunohistochemistry for Hsf-1 and 1C2 in the cerebral motor cortex of AR-97Q and Hsf-1 -knockout AR-97Q mice (13 weeks old). In AR-97Q mice, 1C2-positive cells were observed in the fifth layer of the cerebral motor cortex, where the expression levels of Hsf-1 were relatively lower than in the other layers. The distribution of pathogenic AR accumulation (red arrows) was expanded to the second and third layers of the cerebral motor cortex in heterozygous Hsf-1 -knockout AR-97Q mice. ( g ) Immunoblotting for AR in wild-type, AR-97Q and Hsf-1 -knockout AR-97Q mice (13 weeks old). Pathogenic AR oligomers are indicated by a smear from the top of the gel. *Nonspecific bands. ( h ) Quantitative analysis of immunoblots using densitometry indicated that the expression levels of abnormal AR protein complexes in the spinal cord, cerebral cortex, striatum and cerebellum were upregulated in heterozygous Hsf-1 -knockout AR-97Q mice compared with AR-97Q mice. ( i ) Quantification of immunoblotting revealed that the expression levels of AR monomer were upregulated in the spinal cord, striatum and cerebellum of heterozygous Hsf-1 -knockout AR-97Q mice. * P <0.05, ** P <0.01 by unpaired t -test. More than 500 neurons from three brains were analysed in each group ( b – e ). Unpaired t -test ( n =3) ( h , i ). Error bars indicate s.e.m. ( b – e , h , i ). Scale bars, 50 μm ( a ). NS, not significant. Full size image Hsf-1 depletion aggravates neurodegeneration in SBMA mice To examine whether the decreased expression levels of Hsf-1 leads to increased motor neuronal damage in the SBMA mouse model, we analysed the effects of Hsf-1 depletion on the neurological and histopathological phenotypes of AR-97Q mice. The results demonstrated that muscle atrophy was enhanced in the Hsf-1 -knockout AR-97Q mice compared with the genetically unmodified AR-97Q mice ( Fig. 4a and Supplementary Movie 1). Footprint analysis showed that the stride length was shortened and the paws were dragged in the heterozygous Hsf-1 -knockout AR-97Q mice ( Fig. 4b ). The heterozygous knockout of Hsf-1 in AR-97Q mice also shortened their lifespan and decreased their body weight, and also exacerbated muscle weakness, as measured using grip power and the rotarod task ( Fig. 4d–g ). To exclude nonspecific effects of Hsf-1 depletion on the motor phenotypes of wild-type mice, we investigated the lifespan and motor function of heterozygous Hsf-1 -knockout wild-type mice ( Supplementary Fig. S5a–d ). The results showed that the heterozygous knockout of Hsf-1 had no influence on the lifespan, body weight or motor function of wild-type mice, suggesting that the deleterious effects of Hsf-1 depletion are disease-specific phenomena. 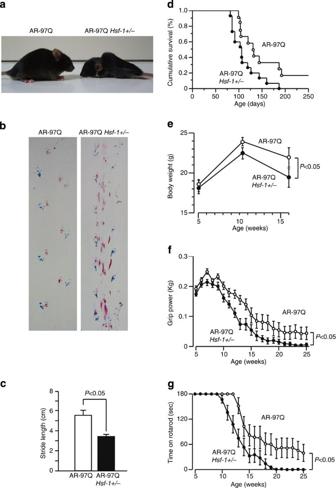Figure 4: HeterozygousHsf-1-knockout AR-97Q mice have more severe muscle atrophy than AR-97Q mice. (a) Muscle atrophy is enhanced in theHsf-1-knockout AR-97Q mice compared with the AR-97Q mice (10 weeks old). (b) Footprints of 13-week-old AR-97Q andHsf-1-knockout AR-97Q mice. The front paws are shown in red, while the hind paws are shown in blue. (c) Quantification of the footprints revealed that the stride length was significantly shortened in the heterozygousHsf-1-knockout AR-97Q mouse (13 weeks old). Unpairedt-test (n=3). Cumulative survival (d), body weight (e), grip power (f) and Rotarod task (g) of AR-97Q andHsf-1-knockout AR-97Q mice. There were significant differences in all parameters between the AR-97Q (n=12) and heterozygousHsf-1-knockout AR-97Q (n=15) mice by unpairedt-test:P<0.05 (d);P<0.05 at 16 weeks (e);P<0.05 at 25 weeks (f); andP<0.05 at 25 weeks (g). Error bars indicate s.e.m. (c–g). Figure 4: Heterozygous Hsf-1 -knockout AR-97Q mice have more severe muscle atrophy than AR-97Q mice. ( a ) Muscle atrophy is enhanced in the Hsf-1 -knockout AR-97Q mice compared with the AR-97Q mice (10 weeks old). ( b ) Footprints of 13-week-old AR-97Q and Hsf-1 -knockout AR-97Q mice. The front paws are shown in red, while the hind paws are shown in blue. ( c ) Quantification of the footprints revealed that the stride length was significantly shortened in the heterozygous Hsf-1 -knockout AR-97Q mouse (13 weeks old). Unpaired t -test ( n =3). Cumulative survival ( d ), body weight ( e ), grip power ( f ) and Rotarod task ( g ) of AR-97Q and Hsf-1 -knockout AR-97Q mice. There were significant differences in all parameters between the AR-97Q ( n =12) and heterozygous Hsf-1 -knockout AR-97Q ( n =15) mice by unpaired t -test: P <0.05 ( d ); P <0.05 at 16 weeks ( e ); P <0.05 at 25 weeks ( f ); and P <0.05 at 25 weeks ( g ). Error bars indicate s.e.m. ( c – g ). Full size image To investigate the neuropathological changes underlying the phenotypic aggravation and the increase of pathogenic 1C2-positive neuronal cells, we performed immunohistochemistry on the spinal anterior horn, cerebral cortex, striatum and cerebellum of heterozygous Hsf-1 -knockout and genetically unmodified AR-97Q mice using antibodies against choline acetyl transferase (ChAT), NeuN and calbindin. The results showed that neurons in each part of the CNS were atrophied in the Hsf-1 -knockout AR-97Q mice ( Fig. 5a–h ). Western blot analysis confirmed the decreased levels of ChAT, a functional marker of spinal motor neurons, in the heterozygous Hsf-1 -knockout AR-97Q mice ( Fig. 5i ). 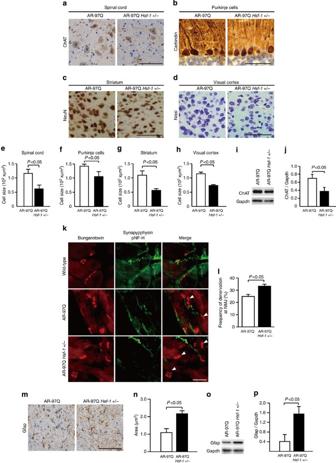Figure 5: Histopathological change in the CNS ofHsf-1-knockout AR-97Q mice. (a–d) Histopathological analyses of AR-97Q andHsf-1-knockout AR-97Q mice (13 weeks old). Immunohistochemistry for ChAT in the anterior horn of the spinal cord (a). Immunohistochemistry for calbindin in Purkinje cells (b). Immunohistochemistry for NeuN in the striatum (c). Nissl staining of the cerebral cortex (d). (e–h) Quantitative analysis of the size of neurons revealed that the neurons in each part of the CNS became atrophied in theHsf-1-knockout AR-97Q mice compared with the AR-97Q mice. (i) Immunoblotting for ChAT in the spinal cord of AR-97Q andHsf-1-knockout AR-97Q mice (13 weeks old). (j) Quantitative analysis of the signal intensity of the ChAT-immunoreactive bands. (k) Immunofluorescent staining of NMJs in 13-week-old AR-97Q and heterozygousHsf-1-knockout AR-97Q mice (red, bungarotoxin; green, synaptophysin and phopsho-neurofilament H).The terminal of motor axons (green) are merged with virtually all the acetylcholine receptors labelled by bungarotoxin (red) in wild-type mice, indicating that NMJs are fully innervated. By contrast, some NMJs of AR-97Q mice lack synaptophysin and phopsho-neurofilament H staining owing to denervation (arrowheads), and this phenomenon was further enhanced byHsf-1depletion. (l) The frequency of denervation at NMJ is significantly increased in heterozygousHsf-1-knockout AR-97Q mice. (m) Immunohistochemistry for Gfap in the anterior horn of the spinal cord. (n) Quantitative analysis of anti-Gfap immunoreactivity. (o) Immunoblotting for Gfap in the spinal cord of AR-97Q andHsf-1-knockout AR-97Q mice (13 weeks old). (p) Quantitative analysis of the signal intensity of the Gfap-immunoreactive bands. Unpairedt-test. More than 500 neurons from three brains were analysed in each group (e–h),n=3 (j). Unpairedt-test.n=3 for each group (l),n=5 (n). Error bars indicate s.e.m. (e–h,j,l,n,p). Scale bars, 50 μm (a–d,k,m). Figure 5: Histopathological change in the CNS of Hsf-1 -knockout AR-97Q mice. ( a – d ) Histopathological analyses of AR-97Q and Hsf-1 -knockout AR-97Q mice (13 weeks old). Immunohistochemistry for ChAT in the anterior horn of the spinal cord ( a ). Immunohistochemistry for calbindin in Purkinje cells ( b ). Immunohistochemistry for NeuN in the striatum ( c ). Nissl staining of the cerebral cortex ( d ). ( e – h ) Quantitative analysis of the size of neurons revealed that the neurons in each part of the CNS became atrophied in the Hsf-1 -knockout AR-97Q mice compared with the AR-97Q mice. ( i ) Immunoblotting for ChAT in the spinal cord of AR-97Q and Hsf-1 -knockout AR-97Q mice (13 weeks old). ( j ) Quantitative analysis of the signal intensity of the ChAT-immunoreactive bands. ( k ) Immunofluorescent staining of NMJs in 13-week-old AR-97Q and heterozygous Hsf-1 -knockout AR-97Q mice (red, bungarotoxin; green, synaptophysin and phopsho-neurofilament H).The terminal of motor axons (green) are merged with virtually all the acetylcholine receptors labelled by bungarotoxin (red) in wild-type mice, indicating that NMJs are fully innervated. By contrast, some NMJs of AR-97Q mice lack synaptophysin and phopsho-neurofilament H staining owing to denervation (arrowheads), and this phenomenon was further enhanced by Hsf-1 depletion. ( l ) The frequency of denervation at NMJ is significantly increased in heterozygous Hsf-1 -knockout AR-97Q mice. ( m ) Immunohistochemistry for Gfap in the anterior horn of the spinal cord. ( n ) Quantitative analysis of anti-Gfap immunoreactivity. ( o ) Immunoblotting for Gfap in the spinal cord of AR-97Q and Hsf-1 -knockout AR-97Q mice (13 weeks old). ( p ) Quantitative analysis of the signal intensity of the Gfap-immunoreactive bands. Unpaired t -test. More than 500 neurons from three brains were analysed in each group ( e – h ), n =3 ( j ). Unpaired t -test. n =3 for each group ( l ), n =5 ( n ). Error bars indicate s.e.m. ( e – h , j , l , n , p ). Scale bars, 50 μm ( a – d , k , m ). Full size image To analyse the effects of Hsf-1 depletion on the denervation at neuromuscular junctions (NMJs) of AR-97Q mice, we performed immunofluorescent staining of NMJs using α-bungarotoxin together with antibodies against synaptophysin and phospho neurofilament ( Fig. 5k ). Quantitative analysis showed that the frequency of denervation at NMJ is increased in the heterozygous Hsf-1 -knockout SBMA mice compared with the AR-97Q mice ( Fig. 5l ). In addition, immunohistochemistry and immunoblot analysis using an antibody against glial fibrillary acid protein (GFAP) showed increased immunoreactivity in the anterior horn of the spinal cord of the heterozygous Hsf-1 -knockout SBMA mice compared with AR-97Q mice, indicating that motor neuron degeneration was enhanced by the partial depletion of Hsf-1 ( Fig. 5m–p ). Furthermore, haematoxylin and eosin staining demonstrated that skeletal muscle fibres were atrophied in the heterozygous Hsf-1 -knockout AR-97Q mice compared with the genetically unmodified AR-97Q mice, suggesting the aggravation of neurogenic amyotrophy ( Supplementary Fig. S6a,b ). Tissue-specific regulation of Hsps in SBMA mice To confirm that the heterozygous knockout of Hsf-1 leads to the downregulation of Hsps, we performed immunoblotting on several tissues from each mouse group. We found that the degree of Hsf-1 downregulation differed in a tissue-specific manner in the heterozygous Hsf-1 -knockout SBMA mice. For example, the protein levels of Hsf-1 were significantly decreased by the heterozygous knockout of Hsf-1 in the spinal cord, liver and skeletal muscle ( Fig. 6a–d ). Conversely, the expression levels of Hsf-1 were not changed in the testis of the heterozygous Hsf-1 -knockout AR-97Q mice compared with the AR-97Q mice ( Fig. 6a ). In accordance with these findings, Hsp72, the inducible form of Hsp70, was downregulated in the spinal cord and liver, but not in the testis, of the heterozygous Hsf-1 -knockout AR-97Q mice ( Fig. 6a–c ). Moreover, Hsp105 was also significantly downregulated in the spinal cord and liver of the heterozygous Hsf-1 -knockout mice ( Fig. 6a–c ). However, the expression levels of Hsps within skeletal muscle were not changed by Hsf-1 depletion ( Fig. 6a ). Similar findings were observed in the heterozygous Hsf-1 -knockout wild-type mice compared with wild-type mice ( Supplementary Fig. S7a–d ). To confirm that the downregulation of Hsp72 following Hsf-1 depletion was via the decrease of messenger RNA levels, we analysed the mRNA expression levels of Hsp70A1 , the gene encoding Hsp72, in the spinal cord, liver and skeletal muscle. The results showed that the mRNA levels of Hsp70A1 were decreased in the spinal cord and liver of the heterozygous Hsf-1 -knockout AR-97Q mice, in agreement with the immunoblotting findings ( Fig. 6f ). In contrast, the heterozygous knockout of Hsf-1 did not alter the mRNA levels of Hsp70A1 in skeletal muscle ( Fig. 6h ). There were no detectable changes in the expression levels of Hsp40 and Hsp90 in all the tissues examined from heterozygous Hsf-1-knockout AR-97Q mice ( Fig. 6a–e ). These findings are compatible with the change in the distribution of pathogenic AR accumulation, and indicate that the induction of Hsp70 is dependent on the expression levels of Hsf-1 in the spinal cord and liver, but not in the skeletal muscle, of the SBMA model mice. 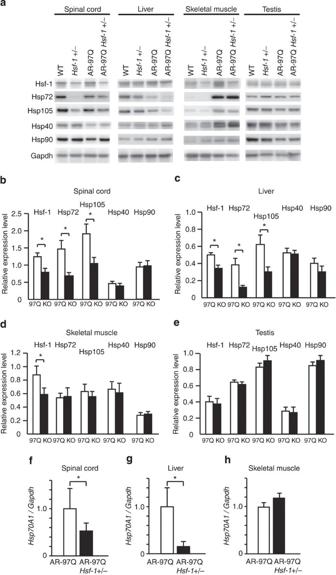Figure 6: Expression levels of Hsps in tissues fromHsf-1-knockout AR-97Q mice. (a) Immunoblotting for Hsf-1, Hsp72, Hsp105, Hsp40 and Hsp90 in wild-type,Hsf-1-knockout wild-type, AR-97Q and Hsf-1-knockout AR-97Q mice (13 weeks old). (b–e) Quantitative analysis using densitometry revealed that the expression levels of Hsp72 in the spinal cord (b) and liver (c) were downregulated in heterozygousHsf-1-knockout AR-97Q mice compared with AR-97Q mice (13 weeks old). No significant alterations in the signal intensity of the Hsp-immunoreactive bands were observed in skeletal muscle (d) or testis (e). Data are shown as the ratio of the intensity of each molecule to Gapdh. (f–h) Quantification ofHsp70A1mRNA levels using RT-PCR in the spinal cord (f), liver (g) and skeletal muscle (h). *P<0.05 by unpairedt-test (n=7) (b–e), and (n=3) (f–h). The inter-group differences were not significant, unless otherwise mentioned. Error bars indicate s.e.m. (b–h). Figure 6: Expression levels of Hsps in tissues from Hsf-1 -knockout AR-97Q mice. ( a ) Immunoblotting for Hsf-1, Hsp72, Hsp105, Hsp40 and Hsp90 in wild-type, Hsf-1 -knockout wild-type, AR-97Q and Hsf-1-knockout AR-97Q mice (13 weeks old). ( b – e ) Quantitative analysis using densitometry revealed that the expression levels of Hsp72 in the spinal cord ( b ) and liver ( c ) were downregulated in heterozygous Hsf-1 -knockout AR-97Q mice compared with AR-97Q mice (13 weeks old). No significant alterations in the signal intensity of the Hsp-immunoreactive bands were observed in skeletal muscle ( d ) or testis ( e ). Data are shown as the ratio of the intensity of each molecule to Gapdh. ( f – h ) Quantification of Hsp70A1 mRNA levels using RT-PCR in the spinal cord ( f ), liver ( g ) and skeletal muscle ( h ). * P <0.05 by unpaired t -test ( n =7) ( b – e ), and ( n =3) ( f – h ). The inter-group differences were not significant, unless otherwise mentioned. Error bars indicate s.e.m. ( b – h ). Full size image To elucidate the molecular machinery underlying the Hsf-1-independent regulation of Hsp70 expression in the skeletal muscle of AR-97Q mice, we investigated the expression levels of several major transcription factors, such as Nfya, Tbp, p53 and Sp1, which also regulate the expression of Hsp70 (refs 18 , 19 , 35 , 36 , 37 ). The results showed that Nfya and Sp1, but not Tbp nor p53, were upregulated in the skeletal muscle of AR-97Q mice compared with wild-type mice ( Fig. 7a ). This upregulation was further enhanced by the partial depletion of Hsf-1 ( Fig.7a–c ). In contrast to the skeletal muscle, neither Nfya nor Sp1 were upregulated by Hsf-1 depletion in the spinal cord or liver of AR-97Q mice ( Fig. 7d ). Immunohistochemical analysis showed an increase in the levels of nuclear Nfya and Sp1 in the skeletal muscle of AR-97Q mice, which was further intensified by the heterozygous knockout of Hsf-1 ( Fig. 7f–h ). These findings suggest that proteins such as Nfya and Sp1 appear to regulate the expression of Hsp70 and this probably underlies the observation that pathogenic AR accumulation was not increased in the skeletal muscle of the Hsf-1 -depleted AR-97Q mice. 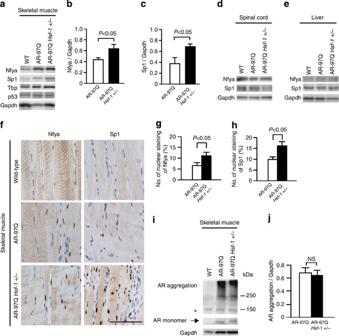Figure 7: Expression levels of Hsp70 inducers in skeletal muscle. (a) Immunoblotting for Nfya, Sp1, p53 and Tbp in wild-type, AR-97Q and heterozygousHsf-1-knockout AR-97Q mice (13 weeks old). (b,c) Quantitative analysis using densitometry revealed that the expression levels of Nfya and Sp1 in skeletal muscle were upregulated in heterozygousHsf-1-knockout AR-97Q mice compared with AR-97Q mice (13 weeks old). (d,e) Immunoblotting for Nfya and Sp1 in the spinal cord and liver in the mice of each group (13 weeks old). (f) Immunohistochemistry of skeletal muscle in wild-type, AR-97Q andHsf-1-knockout AR-97Q mice using anti-Nfya and anti-Sp1 antibodies (13 weeks old). The nuclear uptake of Nfya and Sp1 was upregulated in AR-97Q mice compared with wild-type mice, and further intensified in heterozygousHsf-1-knockout AR-97Q mice. (g,h) Quantification of immunohistochemistry with Nfya and Sp1 in the skeletal muscle of heterozygousHsf-1-knockout AR-97Q mice compared with AR-97Q mice (13 weeks old). (i) Immunoblotting for AR in wild-type, AR-97Q andHsf-1-knockout AR-97Q mice (13 weeks old). *Nonspecific bands. Quantitative analysis of immunoblots using densitometry indicated that the expression levels of abnormal AR aggregations in the skeletal muscle had no significant change in heterozygousHsf-1-knockout AR-97Q mice compared with AR-97Q mice (j). Unpairedt-test (n=3). Error bars, s.e.m. (b,c,g,h,j). Scale bars, 50 μm (f). NS, not significant. Figure 7: Expression levels of Hsp70 inducers in skeletal muscle. ( a ) Immunoblotting for Nfya, Sp1, p53 and Tbp in wild-type, AR-97Q and heterozygous Hsf-1 -knockout AR-97Q mice (13 weeks old). ( b , c ) Quantitative analysis using densitometry revealed that the expression levels of Nfya and Sp1 in skeletal muscle were upregulated in heterozygous Hsf-1 -knockout AR-97Q mice compared with AR-97Q mice (13 weeks old). ( d , e ) Immunoblotting for Nfya and Sp1 in the spinal cord and liver in the mice of each group (13 weeks old). ( f ) Immunohistochemistry of skeletal muscle in wild-type, AR-97Q and Hsf-1 -knockout AR-97Q mice using anti-Nfya and anti-Sp1 antibodies (13 weeks old). The nuclear uptake of Nfya and Sp1 was upregulated in AR-97Q mice compared with wild-type mice, and further intensified in heterozygous Hsf-1 -knockout AR-97Q mice. ( g , h ) Quantification of immunohistochemistry with Nfya and Sp1 in the skeletal muscle of heterozygous Hsf-1 -knockout AR-97Q mice compared with AR-97Q mice (13 weeks old). ( i ) Immunoblotting for AR in wild-type, AR-97Q and Hsf-1 -knockout AR-97Q mice (13 weeks old). *Nonspecific bands. Quantitative analysis of immunoblots using densitometry indicated that the expression levels of abnormal AR aggregations in the skeletal muscle had no significant change in heterozygous Hsf-1 -knockout AR-97Q mice compared with AR-97Q mice ( j ). Unpaired t -test ( n =3). Error bars, s.e.m. ( b , c , g , h , j ). Scale bars, 50 μm ( f ). NS, not significant. Full size image To investigate the effects of Hsf-1 on the pathogenic AR aggregations in the skeletal muscle, we analysed immunoblots of the tissue using an anti-AR antibody. The results showed that the amount of oligomers or monomer of pathogenic AR was not increased by the heterozygous depletion of Hsf-1 in the skeletal muscle of AR-97Q mice ( Fig. 7i ). In agreement with these immunoblot analyses, immunohistochemistry demonstrated no significant difference in the number of 1C2-positive cells in the skeletal muscle between the heterozygous Hsf-1 -knockout and genetically unmodified AR-97Q mice ( Supplementary Fig. S8a,b ). Overexpression of Hsf-1 suppresses AR accumulation To investigate whether Hsf-1 exerts neuroprotection in the mouse model of SBMA, we administered a lentiviral vector expressing green fluorescent protein (GFP) with or without human HSF-1 into the motor cortex and striatum of the AR-97Q mice ( Fig. 8a ), as previous reports showed that no line of transgenic mice of HSF-1 demonstrates an increased expression level of this protein in the brain [38] . We performed stereotaxic injection of the lentiviral vector into the motor cortex or striatum of 8-week-old SBMA mice. Three weeks after the surgery, neuronal size and frequency of abnormal AR accumulation were examined. In both the motor cortex and striatum, the frequency of pathogenic AR accumulation around the lentiviral vector-injected area where HSF-1 was highly expressed was decreased in comparison with that in the contralateral side without treatment ( Fig. 8b ). In addition, the neuron sizes of the motor cortex and striatum were significantly increased by the HSF-1 injecteion ( Fig. 8b ). Quantitative analyses confirmed these findings, whereas the lentiviral delivery of GFP without HSF-1 failed to show any neuroprotective effects ( Fig. 8c–e and Supplementary Fig. S9a–j ). These results indicated that HSF-1 overexpression attenuated the accumulation of pathogenic AR and eventual neurodegeneration in the brain of the SBMA mice. 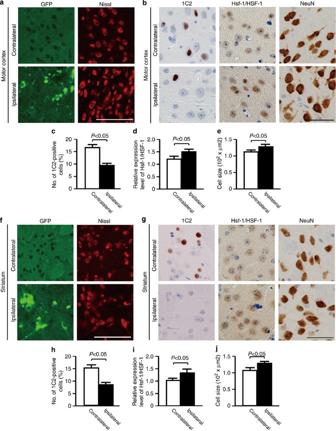Figure 8: HSF-1 alleviates neuronal atrophy in the motor cortex and striatum of AR-97Q mice. (a,f) Expression of transgenes in the motor cortex (a) and striatum (f) of the AR-97Q mice 3 weeks after injection. (b,g) Immunohistochemistry for Hsf-1/HSF-1, 1C2 and NeuN in the motor cortex and striatum of AR-97Q mice. The regions injected with lentiviral vector expressing hHSF-1 were compared with the contralateral side of the same mouse (13 weeks old). (c–e,h–j) Quantitative analyses of the frequency of 1C2-positive cells (c,h), relative expression level of Hsf-1/HSF-1 (d,i) and cell size of neuronal cells (e,j) confirmed the neuroprotection by the lentiviral delivery of HSF-1 into the motor cortex and striatum of AR-97Q mice. Unpairedt-test. More than 300 neurons from three brains were analysed in each group (c–e,h–j). Error bars indicate s.e.m. (c–e,h–j). Scale bars, 100 μm (a,f) and 50 μm (b,g). Figure 8: HSF-1 alleviates neuronal atrophy in the motor cortex and striatum of AR-97Q mice. ( a , f ) Expression of transgenes in the motor cortex ( a ) and striatum ( f ) of the AR-97Q mice 3 weeks after injection. ( b , g ) Immunohistochemistry for Hsf-1/HSF-1, 1C2 and NeuN in the motor cortex and striatum of AR-97Q mice. The regions injected with lentiviral vector expressing hHSF-1 were compared with the contralateral side of the same mouse (13 weeks old). ( c – e , h – j ) Quantitative analyses of the frequency of 1C2-positive cells ( c , h ), relative expression level of Hsf-1/HSF-1 ( d , i ) and cell size of neuronal cells ( e , j ) confirmed the neuroprotection by the lentiviral delivery of HSF-1 into the motor cortex and striatum of AR-97Q mice. Unpaired t -test. More than 300 neurons from three brains were analysed in each group ( c – e , h – j ). Error bars indicate s.e.m. ( c – e , h – j ). Scale bars, 100 μm ( a , f ) and 50 μm ( b , g ). Full size image In summary, we showed that the expression level of Hsf-1 influences the nuclear accumulation of pathogenic AR, and that the depletion of this transcription factor leads to the expanded distribution of pathological lesions and phenotypic exacerbation in the SBMA mouse model. However, these phenomena were not observed in skeletal muscle, where alternative regulators of Hsps, such as Nfya and Sp1, were upregulated. In addition, exogenous overexpression of HSF-1 using a lentivirus vector protected the neurons within the susceptible lesions of SBMA mice. Our results suggest that Hsf-1 contributes to the pathological lesion selectivity in SBMA, and that the tissue-specific regulation of Hsps should be taken into account for the development of therapies that induce the expression of molecular chaperones. In the present study, the heterozygous knockout of Hsf-1 substantially augmented the nuclear accumulation of pathogenic AR in the CNS, suppressed the intraneuronal expression of Hsp70, diminished the size of affected neurons and exacerbated the neurological symptoms in a mouse model of SBMA. By contrast, the lentiviral delivery of HSF-1 attenuated pathogenic AR accumulation and neuronal atrophy in the brain of the SBMA mice. Hsps, particularly Hsp70, have a protective role in neurodegeneration by preventing the accumulation of abnormal proteins [4] , [39] , [40] , [41] , [42] , [43] . However, the role of Hsf-1 in the induction of Hsps is controversial in experiments using cellular models of polyglutamine diseases [18] , [19] , [38] , [44] . The results of the present study demonstrate that the expression of Hsp70, but not Hsp40, is regulated by Hsf-1 in various neurons including spinal motor neurons in the SBMA mouse model. As for the neuroprotective properties of Hsf-1 against cellular stresses, several studies showed that the overexpression of Hsf-1 suppresses the toxicity of polyglutamine-expanded proteins in cultured cells and rodents [38] , [44] . The present study also demonstrated the neuroprotective effects of the exogenous HSF-1 in the CNS of SBMA model mice. By contrast, the depletion of Hsf-1 shortens the lifespan of a mouse model of HD, although the associated histopathological and biochemical alterations were not thoroughly examined [33] . Taken together, our findings indicate that the Hsf-1–Hsp70 pathway exerts neuroprotective effects via the suppression of pathogenic protein accumulation in the pathogenesis of polyglutamine-induced neurodegeneration. The most intriguing finding of the present study is that the heterozygous depletion of Hsf-1 altered the histopathological distribution of pathogenic AR accumulation in the AR-97Q mice, indicating a role for Hsf-1 in the selectivity of the pathogenic lesions in SBMA. The selective damage of specific subgroups of neuronal and non-neuronal cells, despite the ubiquitous expression of the causative protein, is a characteristic of neurodegenerative diseases, although the molecular mechanisms underlying this phenomenon remain unclear [23] . In patients with SBMA, the accumulation of pathogenic AR in each tissue corresponds to their clinical symptoms and findings, for example, lower motor neurons for muscle weakness and atrophy, and the pancreas for diabetes. Nevertheless, the distribution of pathogenic AR accumulation is not equivalent to the expression pattern of normal AR [20] , [32] . Furthermore, the accumulation of pathogenic AR is observed in specific tissues of the AR-97Q mice, although the expression of the transgene, which was regulated by a potent chicken-β-actin promoter, was also detected in tissues that showed no histopathological abnormalities [25] , [45] . These findings suggest that factors other than the transcription of mutant AR may contribute to the tissue-specific accumulation of the causative protein. In the present study, the heterozygous knockout of Hsf-1 induced pathogenic AR accumulation in the cerebral visual cortex, liver and pituitary gland, which were not affected in genetically unmodified AR-97Q mice. In addition, the reduction of Hsf-1 expression in hepatocytes resulted in the exacerbation of liver dysfunction and cellular atrophy in the SBMA mouse model. Given that the defect of protein turnover leads to cellular atrophy [46] , the impairment of protein quality control due to pathological AR accumulation induced by Hsf-1 depletion may underlie the hepatocyte atrophy [47] . These findings indicate that endogenous Hsf-1 can clear certain lesions, such as in the cerebral visual cortex, liver and pituitary gland, of pathogenic AR accumulation and that the expression levels of Hsf-1 in each tissue, at least partially, influence the pathogenic lesion selectivity of SBMA. The results of the present study also revealed the tissue-specific regulation of Hsps by Hsf-1. Despite downregulation of Hsps in spinal cord and liver, Hsf-1 depletion had no effect on the expression of Hsps in the testis of AR-97Q mice, presumably owing to an incomplete reduction of Hsf-1 protein levels. Furthermore, the inactivation of Hsf-1 did not decrease the expression levels of Hsps or enhance the accumulation of pathogenic AR in the skeletal muscle of SBMA mice, suggesting that molecules other than Hsf-1 may maintain the expression of Hsps. The upregulation of Nfya and Sp1 in the skeletal muscle of the heterozygous Hsf-1 -knockout AR-97Q mice appears to compensate for the deleterious effects of Hsf-1 depletion on the transcriptional regulation of Hsp70, given that these molecules are capable of inducing the expression of Hsps in certain circumstances [36] , [37] , [48] . In contrast, this compensatory mechanism does not function in the spinal cord, providing another molecular basis for the vulnerability of motor neurons in SBMA. In support of our findings, a cell-specific compensatory mechanism was shown to influence the selectivity of pathogenic lesions in a mouse model of HD [49] . As Hsf-1 is known to have diverse functions in healthy and disease conditions, such as longevity and inflammation [50] , [51] , further study is needed to thoroughly understand the entire effects of Hsf-1 depletion on the pathogenesis of neurodegenerative diseases. From the therapeutic point of view, the manipulation of tissue-specific regulatory systems of Hsps may be a key strategy to combat the toxicity of polyglutamine-expanded proteins. Animals AR-97Q mice were generated by using the pCAGGS vector and maintained as described previously [25] , [40] . The AR-97Q and heterozygous Hsf-1 -knockout AR-97Q mice, as well as the heterozygous Hsf-1 -knockout wild-type and wild-type mice used in the experiments described here, were derived by crossing heterozygous Hsf-1 -knockout C57BL6 mice with AR-97Q mice [33] . All of the experiments were performed on male mice derived from the cross described above. The mice were genotyped by PCR on tail DNA [25] , [33] . Behavioural analysis All of the tests were performed weekly, and the data were analysed prospectively as described in Supplementary Methods . All of the animal experiments were performed in accordance with the National Institutes of Health Guide for the Care and Use of Laboratory Animals and under the approval of the Nagoya University Animal Experiment Committee. Autopsy specimens Autopsy specimens of the CNS, including the spinal cord, cerebrum and cerebellum, and non-neuronal tissues, such as the pancreas, spleen and colon, were obtained from three genetically confirmed SBMA patients (52, 77 and 78 years old) and three control subjects (58, 64 and 70 years old). Representative sections are shown in Supplementary Fig. S2 . The collection of tissues and their use for this study were approved by the Ethics Committee of Nagoya University Graduate School of Medicine. Immunoblotting Mouse tissues were homogenized in buffer containing 50 mM Tris–HCl (pH 8.0), 150 mM NaCl, 1% Nonidet P-40, 0.5% deoxycholate, 0.1% SDS and 1 mM 2-mercaptoethanol with 1 mM phenylmethylsulphonyl fluoride and 6 μg ml −1 aprotinin and then centrifuged at 2,500 g for 15 min. Equal amounts of protein were separated by 5–20% SDS/PAGE and transferred to Hybond-P membranes (GE Healthcare, Piscataway, NJ, USA). The primary antibodies and their dilutions were as follows: AR (N20, 1:1,000; Santa Cruz Biotechnology, Santa Cruz, CA, USA), Hsp72 (1:1,000; Stressgen Biotechnologies, Victoria, Canada), Hsp40 (1:5,000; Stressgen), Hsp90 (1:1,000; Stressgen), Hsp105 (1:250; Novocastra Laboratories, Newcastle, UK), Hsf-1 (1:5,000; Stressgen), ChAT (1:1,000; Millipore, Billerica, MA, USA), NF-YA (G-2, 1:500; Santa Cruz Biotechnology), SP1 (PEP2, 1:2,000; Santa Cruz Biotechnology), TBP (N-12, 1:500; Santa Cruz Biotechnology) and p53 (DO-1, 1:500, Santa Cruz Biotechnology). Primary antibody binding was probed with horseradish peroxidase-conjugated secondary antibodies at a dilution of 1:5,000, and bands were detected by using an immunoreaction-enhancing solution (Can Get Signal; Toyobo, Osaka, Japan) and enhanced chemiluminescence (ECL Plus; GE Healthcare). An LAS-3000 imaging system (Fujifilm, Tokyo, Japan) was used to produce digital images. The signal intensities of these independent blots were quantified using IMAGE GAUGE software version 4.22 (Fuji) and expressed in arbitrary units. The membranes were reprobed with an anti-GAPDH (1:5,000; Santa Cruz Biotechnology) antibody for normalization. Histology and immunohistochemistry Mice deeply anesthetized with pentobarbital were perfused with 4% paraformaldehyde fixative in phosphate buffer (pH 7.4). The tissues were dissected, post-fixed in 10% phosphate-buffered formalin and processed for paraffin embedding. Sections to be stained with an anti-polyglutamine antibody (1C2) were treated with formic acid for 5 min at room temperature; those to be incubated with an anti-HSF-1 antibody were boiled in 10 mM citrate buffer for 15 min. The primary antibodies and their dilutions were as follows: polyglutamine (1:20,000; Millipore), Hsp72 (1:500; Stressgen), anti-HSF-1 (1:5,000; Stressgen), ChAT (1:1,000; Millipore), GFAP (1:2,000; Epitomics, Burlingame, CA, USA), NF-YA (H-209, 1:500; Santa Cruz Biotechnology), SP1 (PEP2, 1:2,000; Santa Cruz Biotechnology), TBP (N-12, 1:500; Santa Cruz Biotechnology), and p53 (DO-1, 1:500; Santa Cruz Biotechnology). Primary antibody binding was probed with a secondary antibody labelled with a polymer as part of the Envision+ system containing horseradish peroxidase (Dako Cytomation, Gostrup, Denmark). Lentiviral vector construct preparation The cds portion of human HSF-1 complementary DNA [33] was subcloned into the pEGFP expression vector through Age1 and Xho1 restriction sites. hHSF-1-GFP was inserted into the pENTR/D/TOPO vector (Invitrogen, Carlsbad, CA) and transferred into the pLenti CMV Neo DEST #2 (705-1) vector, a gift from Dr Eric Campeau (Resverlogix Corp.), using the Gateway system (Invitrogen). Viral production Lentivirus was prepared following Campeu’s protocol [52] . Briefly, lentiviral particles were produced in HEK293FT cells by transfection using Lipofectamine 2000 (Invitrogen). The lentiviral-containing supernatant was collected 48 h after transfection, and concentrated by ultracentrifugation. The viral titre was measured using Lenti-X qRT-PCR Titration Kit (Clontech, Mountain View, CA). Injection procedures Recombinant lentiviral vector expressing hHSF1-GFP or GFP alone (6.7 × 10 8 copies per μl) was stereotaxically injected into the right motor cortex and striatum (1 μl per 10 min) of 8-week-old AR-97Q mice deeply anethetized with pentobarbital, using a Hamilton syringe (Hamilton, Reno, NV, USA) and a microinjection cannula (Eicom, Kyoto, Japan) as described in Supplementary Method . Quantitative analysis of immunohistochemistry To assess 1C2-positive cells, we prepared at least 100 consecutive 6-μm-thick axial sections of the thoracic spinal cord, coronal sections of the cerebrum and cerebellum, and longitudinal sections of skeletal muscle, and immunostained every tenth section with an anti-1C2 antibody. The number of 1C2-positive cells was counted in all of the motor neurons within the anterior horn of the ten axial sections from the thoracic spinal cord and more than 500 neurons in five randomly selected X400 microscopic fields of the ten sections in each region from the cerebrum and cerebellum of each group of mice ( n =3) under a light microscope (Bx51; Olympus, Tokyo, Japan). The frequency of 1C2-positive cells was expressed as the number per 100 neurons. For the assessment of 1C2-positive cells in skeletal muscle, the number of 1C2-positive cells was calculated for more than 500 fibres in randomly selected areas of the ten axial sections and the results were expressed as the number per 100 muscle fibres. To measure the number of 1C2-positive cells in the liver and pituitary gland, more than 500 cells in randomly selected areas of the ten axial sections were investigated and the results were expressed as the number per 100 cells. For the quantification of the expression levels of Hsf-1, Nfya, p53, Tbp and Sp1, we performed immunohistochemistry on every 20th section from the 100 consecutive sections. We measured the intensity of nuclear immunoreactivity for each molecule in the anterior horn of the five axial sections from the thoracic spinal cord and more than 500 cells in five randomly selected X400 microscopic fields of the five sections from the cerebral motor and visual cortex, striatum, and cerebellar Purkinje and granule cells from each group of mice ( n =3) using an image analyser (WinROOF; Mitani Corporation, Tokyo, Japan). We also measured the intensity of immunoreactivity in the ependymal cells of each section as a standard control, and calculated the signal intensity ratio using this control. To quantify the cell size of motor neurons and the region of anti-GFAP immunoreactivity in the spinal anterior horn, we analysed every tenth section of the 50 consecutive 6-μm-thick axial sections from the thoracic spinal cord using an image analyser (WinROOF). For the purposes of calculating the cell size of hepatocytes, cerebellar Purkinje cells, striatal neurons and cerebral cortex neurons, more than 500 neurons and 1000 hepatocytes in randomly selected areas were examined using an image analyser (WinROOF). To analyse the pathological change in the brain with the lentivirus injection, we prepared consecutive 3-μm-thick coronal sections of the cerebrum and immunostained every five sections with 1C2 and anti-Hsf-1 antibodies. The number of 1C2-positive cells was counted in more than 300 neurons in a X400 microscopic fields around the lentivirus injection site from the five sections under a light microscope (Bx51; Olympus, Tokyo, Japan). We measured the intensity of nuclear immunoreactivity for Hsf-1 in more than 300 cells in X400 microscopic fields using an image analyser (WinROOF). NMJ staining 30 μm-thick frozen longitudinal sections of the gastrocnemius muscle were incubated overnight with α-bungarotoxin conjugated with biotinXX (1:80, Invitrogen), anti-phosphorylated NF-H mouse monoclonal antibody (SMI31, 1:100, Covance) and anti-synaptophysin rabbit polyclonal antibody (1:100, Cell Signaling Technologies). After washing, sections were incubated with goat anti-rabbit and anti-mouse IgG conjugated with Alexa 488 (1:1,000 for each, Invitrogen) and streptavidin conjugated with Alexa 564 (1:1,000, Invitrogen) and mounted with Prolong gold (Invitrogen). The stained sections were imaged with an upright microscope (Axio Imager M1, Zeiss). More than 50 NMJs from AR-97Q and heterozygous Hsf-1-knockout AR-97Q mice (13 weeks old) were analysed ( n =3). Quantitative real-time reverse transcriptase PCR (RT–PCR) The mRNA levels of Hsp70A1 were analysed by real-time RT-PCR as described previously [41] . Detailed methods are described in Supplementary Methods . Statistical analysis We analysed the data by using the unpaired Student’s t -test for two group comparisons, and the Kaplan–Meier and log-rank tests for survival rate using STATVIEW software version 5 (Hulinks, Tokyo, Japan), and denoted P -values of 0.05 or less as statistically significant. How to cite this article: Kondo, N. et al . Heat shock factor-1 influences pathological lesion distribution of polyglutamine-induced neurodegeneration. Nat. Commun. 4:1405 doi: 10.1038/ncomms2417 (2013).